One hundred fold increase in current carrying capacity in a carbon nanotube–copper composite Increased portability, versatility and ubiquity of electronics devices are a result of their progressive miniaturization, requiring current flow through narrow channels. Present-day devices operate close to the maximum current-carrying-capacity (that is, ampacity) of conductors (such as copper and gold), leading to decreased lifetime and performance, creating demand for new conductors with higher ampacity. Ampacity represents the maximum current-carrying capacity of the object that depends both on the structure and material. Here we report a carbon nanotube–copper composite exhibiting similar conductivity (2.3–4.7 × 10 5 S cm −1 ) as copper (5.8 × 10 5 S cm −1 ), but with a 100-times higher ampacity (6 × 10 8 A cm −2 ). Vacuum experiments demonstrate that carbon nanotubes suppress the primary failure pathways in copper as observed by the increased copper diffusion activation energy ( ∼ 2.0 eV) in carbon nanotube–copper composite, explaining its higher ampacity. This is the only material with both high conductivity and high ampacity, making it uniquely suited for applications in microscale electronics and inverters. Development of electronic devices is undergoing a paradigm shift with their continued miniaturization [1] . Such miniaturization provides greater portability and versatility to the devices, leading to their ubiquity. Simultaneously, the functionality and performance of these devices have been increasing. Although single-atom transistors [2] and few-atom memory devices [3] have been demonstrated to keep pace with the progressive miniaturization, there has been very little progress in conductors (such as Cu and Au), which supply power to these components within devices. With shrinking size of devices, pathways for carrying current to operate these components have significantly reduced. This has resulted in higher current density being carried by the conductors, reaching the limit of conventional conductors (such as Cu and Au) in present-day devices. In fact, the International Technology Roadmap for Semiconductors (ITRS) predicts [4] that the current density in these devices is expected to exceed the breakdown limit of Cu and Au in 2015. Therefore, new conductors with higher ampacity are in great demand [1] . Ampacity represents the maximum current-carrying capacity of the object that depends both on the structure and material. However, high ampacity and high conductivity are mutually exclusive properties. This is because the former requires a strongly bonded system, whereas the latter requires the free electrons from a weakly bonded system [5] . Therefore, achieving high electrical conductivity and ampacity in the same material has been impossible. Here we report a carbon nanotube–copper (CNT–Cu) composite that overcomes this mutual exclusivity to achieve an ampacity (630 × 10 6 A cm −2 ) 100 times higher than common electrical conductors, such as Cu [6] , [7] , [8] , [9] and Au [9] , [10] ( ∼ 10 6 A cm −2 ), approaching the theoretical limit for CNTs [11] , [12] , [13] , [14] , [15] , [16] (1000 × 10 6 A cm −2 ). Compared with copper, the macroscopic CNT–Cu conductivity (4.7 × 10 5 S cm −1 ) rivaled, exceeded and doubled at 23 °C, above 80 °C and 227 °C, respectively from a one-order-of-magnitude lower temperature coefficient of resistivity. To understand the high ampacity of CNT–Cu composite, we performed activation energy ( E a ) analysis to evaluate the energy required for Cu diffusion in CNT–Cu composite. Our analysis demonstrated that the E a for Cu diffusion in the composite was ∼ 2.0 eV. In comparison, the primary electromigration failure pathways in pure Cu have much lower E a , with surface and grain-boundary Cu diffusion requiring ∼ 0.6 eV and ∼ 1.0 eV, respectively [17] . Thus, the primary electromigration failure pathways (surface and grain-boundary diffusion) are suppressed by the presence of CNTs. Further, Cu diffusion is thus smaller (10 4 times) in our composite compared with bulk Cu, explaining its high ampacity. Conductivity of CNT–Cu composite Significantly, a macroscopic (2.5 × 3.5 cm; Fig. 1a ) CNT–Cu composite solid exhibited a room temperature conductivity of 4.7±0.3 × 10 5 S cm −1 , as measured by the four-probe method, comparable to that of Cu [18] (5.8 × 10 5 S cm −1 ), three orders higher than pristine CNT [19] , [20] ( ∼ 10 2 S cm −1 ) and an order higher than pure CNT fibre [21] (10 4 S cm −1 ). A microscopic CNT–Cu composite fabricated in an identical protocol ( Fig. 1b ) exhibited a room temperature conductivity of 2.1±0.3 × 10 5 S cm −1 . High CNT volume fraction (45 vol%) resulted in a 42% density reduction (5.2 g cm −3 ) compared with Cu [18] (8.9 g cm −3 ). Therefore, the specific conductivity for our CNT–Cu composite was 26% higher than Cu and exceeded most materials (Au, Ag and Cu) with the exception of Al ( Fig. 1j ). The temperature dependence of the conductivity, that is, temperature coefficient of resistivity, of the CNT–Cu composite (7.5 × 10 −4 K −1 ) was one order of magnitude lower than that of Cu [22] (6.8 × 10 −3 K −1 ) ( Fig. 1i ), highlighting one benefit of our CNT–Cu composite. Consequently, the decrease in conductivity with temperature for the CNT–Cu was far less than Cu, and the conductivity was on par at room temperature, exceeded above 80 °C, and was double at 227 °C. This feature is important for heavy load applications, because the operating temperature is often higher than 80 °C. 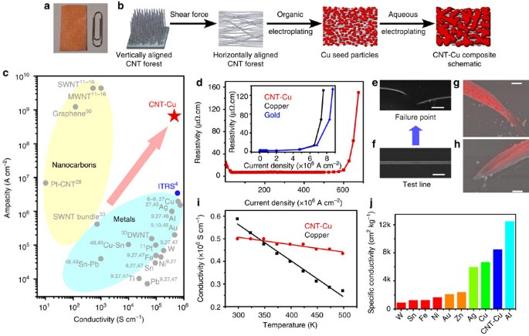Figure 1: Fabrication and ampacity of CNT–Cu composite. (a) Picture of CNT–Cu composite alongside a paperclip for size reference. (b) Schematic representation of various steps for CNT–Cu composite fabrication. Cu seeds nucleate on the CNT surface during the organic electrodeposition and subsequently grow during the aqueous electrodeposition to yield the CNT–Cu composite. (c) Ashby plot of ampacity versus conductivity for various relevant materials, including metals (such as Cu, Au, Ag, Al, etc), alloys (such as Sn-Pb), nanocarbons (such as SWNT, graphene) and composites (such as Pt–CNT). The ITRS recommended level of current density is also shown for comparison, with the performance of CNT–Cu exceeding it. (d) Variation of resistivity with current density for CNT–Cu composite. The electrical conductivity of the wire was 2 × 105S cm−1. Similar traces for Cu and Au lines are shown in inset for comparison. (e) SEM image of CNT–Cu test structure after failure. Scale bar, 4 μm. (f) SEM image of the same CNT–Cu composite test line before failure. Scale bar, 4 μm. (g,h) EDX mapping (based on Cu) of the failure points of CNT–Cu composite line presented inFig. 1e. Scale bar, 500 nm. (i) Variation of conductivity with temperature for CNT–Cu (red) and Cu (black), showing the largely invariant conductivity of CNT–Cu composite with temperature. In comparison, Cu shows a decreasing conductivity with temperature, as expected for metals. (j) Comparison of conductivity per unit weight (specific conductivity) of CNT–Cu with different metals. Figure 1: Fabrication and ampacity of CNT–Cu composite. ( a ) Picture of CNT–Cu composite alongside a paperclip for size reference. ( b ) Schematic representation of various steps for CNT–Cu composite fabrication. Cu seeds nucleate on the CNT surface during the organic electrodeposition and subsequently grow during the aqueous electrodeposition to yield the CNT–Cu composite. ( c ) Ashby plot of ampacity versus conductivity for various relevant materials, including metals (such as Cu, Au, Ag, Al, etc), alloys (such as Sn-Pb), nanocarbons (such as SWNT, graphene) and composites (such as Pt–CNT). The ITRS recommended level of current density is also shown for comparison, with the performance of CNT–Cu exceeding it. ( d ) Variation of resistivity with current density for CNT–Cu composite. The electrical conductivity of the wire was 2 × 10 5 S cm −1 . Similar traces for Cu and Au lines are shown in inset for comparison. ( e ) SEM image of CNT–Cu test structure after failure. Scale bar, 4 μm. ( f ) SEM image of the same CNT–Cu composite test line before failure. Scale bar, 4 μm. ( g , h ) EDX mapping (based on Cu) of the failure points of CNT–Cu composite line presented in Fig. 1e . Scale bar, 500 nm. ( i ) Variation of conductivity with temperature for CNT–Cu (red) and Cu (black), showing the largely invariant conductivity of CNT–Cu composite with temperature. In comparison, Cu shows a decreasing conductivity with temperature, as expected for metals. ( j ) Comparison of conductivity per unit weight (specific conductivity) of CNT–Cu with different metals. Full size image Ampacity of CNT–Cu composite Central to this report, we found that our CNT–Cu exhibited a 100 times higher ampacity than Cu [6] , [7] , [8] , [9] . For this measurement, a CNT–Cu composite line structure (width=800 nm, height=900 nm, length=50 μm) was fabricated by electrodepositing Cu into a CNT line fabricated with conventional electron-beam lithography and reactive ion etching from a thin, closely packed and aligned CNT film [23] , [24] , that is, ‘CNT wafer’. Similar structures with Cu and Au were used for comparison. The current was increased while monitoring the resistivity ( Fig. 1d ). Initially, the resistivity unexpectedly decreased with current. Scanning electron microscopy (SEM) images revealed a smoothening of the initially rough CNT–Cu surface, indicating reorganization of the deposited Cu ( Supplementary Fig. S1 ). We believe that this phenomenon is similar to filament aging to increase lifetime, which contributed to the higher ampacity. The resistivity remained unchanged up to 600 × 10 6 A cm −2 (600 MA cm −2 ), after which the resistivity exponentially increased leading to failure at ∼ 690 MA cm −2 at the central region of the test structure ( Fig. 1e ). The ampacity is defined as the maximum current density where the resistivity remains constant and thus was estimated to be 600 MA cm −2 from an average of five measurements. For comparison, we measured the ampacity of Cu and Au (both wire and sputter-deposited) test structures, which showed ampacities of 6.1 MA cm −2 and 6.3 MA cm −2 , respectively, close to literature values [6] , [7] , [8] , [9] , [10] ( ∼ 1 MA cm −2 ) ∼ 100 times smaller than that of the CNT–Cu composite (inset, Fig. 1d ). Not only was the ampacity of CNT–Cu composite 100 times higher than conventional conductors, such as Cu, Al, Au and Ag [6] , [7] , [8] , [9] , [10] , [25] ( ∼ 1 MA cm −2 ) and reports using Pt decorated CNTs [26] (7.5 MA cm −2 ), it approached the highest value (1,000 MA cm −2 ) reported from individual CNTs [11] , [12] , [13] , [14] , [15] , [16] . Further, the composite was stable at a DC current density of 100 MA cm −2 for over 1200, h (50 days) with less than 10% variation in resistivity ( Supplementary Fig. S2 ). SEM observation of the failure point revealed thinning at both ends of the rupture ( Fig. 1e ). Energy dispersive X-ray microscopy (EDX) detected only carbon at the ruptured surfaces ( Fig. 1g ). These results demonstrate that Cu had diffused away from this region and that the failure mechanism of the CNT–Cu composite was Cu electromigration [27] , [28] , [29] . The CNT–Cu composite was plotted onto a conductivity-ampacity Ashby map for comparison with other high-performance materials ( Fig. 1c ). An inverse trend between conductivity and ampacity was clearly apparent with metals possessing higher conductivities and nanocarbons possessing higher ampacities. The CNT–Cu composite did not follow this trend creating a distinct and isolated point in the high-ampacity and high-conductivity domain with conductivity 1,000 times higher than nanocarbons and ampacity 100 times higher than metals. Although having been proposed theoretically [30] , no methods, to date, have achieved simultaneous increase in both properties. For example, alloying of copper decreases conductivity and doping or bundling of CNTs decreases ampacity [31] . For example, Xu et al . [32] have demonstrated a similar conductivity (no estimation on ampacity) for CNT fibre–Cu composite, but the Cu deposition was limited to the outer surface of the CNT fibre. In this case, the high conductivity is derived from the surface Cu, but we expect that it will fail to exhibit high ampacity. Furthermore, Behabtu et al . [21] reported high conductivity of 2.9 × 10 4 S cm −1 in pure CNT fibre; however, this report also did not characterize the ampacity. Fabrication and characterization of CNT–Cu composite To fabricate a CNT–Cu composite ( Fig. 1a ) that synergistically combines the strengths of both materials, we developed a unique fabrication process. In contrast to conventional approaches that use CNT–Cu ion dispersions, we electrodeposited Cu into the pores of premade, macroscopic CNT structures, for example, buckypaper, and CNT solids (bulk, packed, aligned CNT material [33] ). Long, vertically aligned single-wall CNT forests (diameter=3 nm, height=500–700 μm, density=0.04 g cm −3 ) were synthesized on a substrate by the water-assisted method [34] . The sparse forests were densified ( ∼ 0.5 g cm −3 ) into closely packed and aligned CNT structure by the liquid densification technique [33] with Cu ions. Then, this CNT structure was transformed into CNT–Cu composite by two-stage nucleation-growth electrodeposition processes ( Fig. 1b ), as described below. Several key processes were developed to achieve this CNT–Cu composite. First, the electrodeposition was separated into two phases: (1) wetting the hydrophobic CNTs with Cu ions in an organic solution to nucleate Cu seeds on CNT surface and (2) grow the Cu seeds in an aqueous solution until all the mesopores were filled. Second, in the organic electrodeposition phase, homogeneous seeding required that the rate-limiting step be the Cu nucleation on the CNTs rather than the Cu ion diffusion through the CNT structure. Therefore, slow deposition rates (1–5 mA cm −2 versus conventional rates [35] of 50–100 mA cm −2 ) were required to electrodeposit Cu throughout the dense CNT matrix, not only on the surface. At low current densities (1–5 mA cm −2 ), Cu homogeneously nucleated throughout the CNT matrix, resulting in high conductivity, high Cu filling-ratio and low specific surface area (an indicator of accessible CNT surface area; Fig. 2a ). In contrast, at high current densities (5–15 mA cm −2 ) Cu deposited only at the outer surfaces of the CNT matrix, resulting in exactly the opposite effect ( Fig. 2a ). Third, annealing in hydrogen ambient reduced the (111), (200) and (220) Cu x O y phases to a pure (111), (200) and (220) Cu phase as seen from X-ray diffraction ( Fig. 2b ). In addition, the Cu particles sintered resulting in an improvement in electrical conductivity from 8.2 × 10 3 to 9.1 × 10 4 S cm −1 ( Fig. 2c ). Finally, through aqueous electrodeposition, the Cu volume fraction was increased, as seen by the steep density increase ( Fig. 2c ). 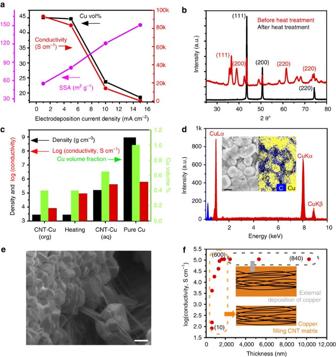Figure 2: Characterization of CNT–Cu composite. (a) Variation of CNT–Cu composite properties as a function of organic electrodeposition current density. The direct correlation between conductivity and volume occupancy of Cu is observed. (b) XRD traces of CNT–Cu composite before (red) and after (black) heat treatment. (c) Evolution of the CNT–Cu composite properties (conductivity, density and Cu volume occupancy) with every advancing step in the fabrication process. Similar properties of bulk Cu are also given alongside for comparison. (d) EDX spectrum of CNT–Cu composite showing the absence of any other impurities with the cross-sectional SEM and EDX mapping images. Scale bar, 2 μm. (e) Cross-sectional SEM images showing the polycrystalline Cu tightly bound with long, intertwined, well-dispersed CNTs. Scale bar, 6 μm. (f) Evolution of CNT–Cu conductivity with thickness and electrodeposition time for a current density of 5 mA cm−2. Values given in brackets pertain to electrodeposition time in minutes. Figure 2: Characterization of CNT–Cu composite. ( a ) Variation of CNT–Cu composite properties as a function of organic electrodeposition current density. The direct correlation between conductivity and volume occupancy of Cu is observed. ( b ) XRD traces of CNT–Cu composite before (red) and after (black) heat treatment. ( c ) Evolution of the CNT–Cu composite properties (conductivity, density and Cu volume occupancy) with every advancing step in the fabrication process. Similar properties of bulk Cu are also given alongside for comparison. ( d ) EDX spectrum of CNT–Cu composite showing the absence of any other impurities with the cross-sectional SEM and EDX mapping images. Scale bar, 2 μm. ( e ) Cross-sectional SEM images showing the polycrystalline Cu tightly bound with long, intertwined, well-dispersed CNTs. Scale bar, 6 μm. ( f ) Evolution of CNT–Cu conductivity with thickness and electrodeposition time for a current density of 5 mA cm −2 . Values given in brackets pertain to electrodeposition time in minutes. Full size image Through this scheme, we succeeded in making a CNT–Cu composite with the CNT covering the surfaces and grain boundaries of Cu (inset, Fig. 2d ). No contamination by oxygen was observed by EDX ( Fig. 2d ). Thermo-gravimetry showed that the composite was composed of ∼ 55 vol% Cu and 45% CNT ( Supplementary Figs S3 and S4 ) (total density=5.2 g cm −3 ), indicating a 42% density reduction from pure Cu [18] (8.9 g cm −3 ). A control experiment was carried out to verify that the observed conductivity arose from the CNT–Cu bulk as opposed to its outer surface. Hence, the thickness and conductivity were plotted as a function of electrodeposition time (10–840 min; Fig. 2f ). Initially (up to 600 min), the electrical conductivity monotonically increased and saturated at 10 5 S cm −1 while the thickness remained unchanged. This meant that the Cu deposited within the CNT matrix. Further electrodeposition (beyond 600 min) led to a thickness increase, which indicated deposition on the outer surfaces. Importantly, the conductivity did not increase during this phase, meaning that the measured conductivity did not stem from the surface deposition of Cu. As experimental results demonstrate, electromigration of Cu atoms is also the failure mechanism of the CNT–Cu composite (like pure Cu). Within this framework, several experiments and analyses were carried out to understand the mechanism of high ampacity of the CNT–Cu composite. The activation energy for Cu diffusion in CNT–Cu composite was estimated by failure kinetics tests carried out at different temperatures (440 K, 450 K, 473 K and 498 K). Applying a current density (720 MA cm −2 ) higher than the ampacity (600 MA cm −2 ) of CNT–Cu results in accelerated failure ( Fig. 3a ). The ‘time of failure,’ t , was estimated from the point of 40% resistivity increase. The results of several such experiments carried out at different temperatures (constant current density) were assembled into an Arrhenius plot of ln( t ) versus 1/kT ( Fig. 3b ). 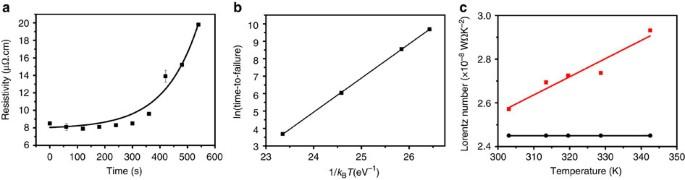Figure 3: Mechanistic analysis of CNT–Cu composite. (a)Variation of resistivity with time for CNT–Cu composite at a current density of 720 MA cm−2at 473 K. (b) Experiment inarepeated at different temperatures to give an Arrhenius plot of ln(time-to-failure) versus 1/kBT. The activation energy for Cu diffusion in CNT–Cu is determined from the slope of this graph. (c) Comparison of Lorentz number for CNT–Cu (red) with Cu (black) as a function of temperature, indicating an increasing phonon contribution of CNT with temperature in CNT–Cu composite. Therefore, the activation energy for Cu diffusion in CNT–Cu composite was estimated from the slope of this plot, based on Black’s equation [36] , Figure 3: Mechanistic analysis of CNT–Cu composite. (a) Variation of resistivity with time for CNT–Cu composite at a current density of 720 MA cm −2 at 473 K. ( b ) Experiment in a repeated at different temperatures to give an Arrhenius plot of ln(time-to-failure) versus 1/ k B T . The activation energy for Cu diffusion in CNT–Cu is determined from the slope of this graph. ( c ) Comparison of Lorentz number for CNT–Cu (red) with Cu (black) as a function of temperature, indicating an increasing phonon contribution of CNT with temperature in CNT–Cu composite. Full size image where j is the current density, E a is the activation energy, k is the Boltzmann constant, T is the mean temperature of the test structure, n is the current-density exponent and A is the pre-exponential factor. The activation energy for Cu diffusion in CNT–Cu composite was estimated, from slope of Fig. 3b to be 2.03 eV. We wish to note that our choice of the current-density exponent ( n ) and pre-exponential factor ( A ) were taken from similar electromigration studies on Cu under identical measurement conditions, namely in vacuum and with the test structure not surrounded by any dielectric [27] , [37] , [38] . Further, we note that this estimation of the activation energy ( E a ) is independent of the choice of pre-exponential factor ( A ) and current-density exponent ( n ). The value of 2.03 eV was identical to that of Cu lattice diffusion [17] , [28] , [29] ( ∼ 2.0–2.3 eV), which means that the Cu diffusion follows the most difficult pathway. For bulk Cu, diffusion occurs at the surfaces and grain boundaries that possess much lower activation energies [17] , [28] , [29] ( ∼ 0.7 eV and ∼ 1.0 eV, respectively). Our results showed that for the CNT–Cu composite, the Cu diffusion pathways through surface and grain boundaries were greatly suppressed. The Cu diffusion coefficient ( D *, related the ease of electromigration) was calculated from the activation energy by: where D 0 is the diffusion coefficient at infinity [17] . As a result, the estimated diffusion coefficient of Cu in the CNT–Cu composite by bulk diffusion was 10 4 times lower than that of copper, which should significantly contribute to the observed high ampacity. Internal structure observations the CNT–Cu composites by SEM and EDX revealed a fine, continuous, mesh-like CNT network covering the surfaces and grain boundaries of Cu (inset, Fig. 2d ). Theoretical studies have proposed that the activation energy for carbon-doped Cu diffusion increased by suppressing surface and grain boundary pathways [39] . Although lowering of Cu electromigration by CNT has been reported, the exact mechanism and the 100 times ampacity increase, without compromising on electrical conductivity, reported here have never been achieved [40] . We draw a distant parallel of this effect with the well-known practice of alloying steel with carbon for strengthening. We believe that the CNT in CNT–Cu composite has a similar role in suppressing Cu diffusion [39] . We numerically estimated the ampacity of the CNT–Cu composite by assuming that the material ruptured by current-induced Joule heating, leading to melting. The temperature increase by current is described by [41] , where j crit is the ampacity, K is the thermal conductivity ( ∼ 800 Wm −1 K −1 ), l is the length of the test structure (50 × 10 −6 m), and L n is the Lorentz number ( ∼ 3.44 × 10 −8 WΩ K −2 ). The melting point of the composite was taken as that of Cu [18] (as 1357 K), because the CNT melting point is significantly higher in an inert ambient. The Lorentz number (ratio of thermal and electrical conductivities) was calculated from the experimentally measured temperature-dependent thermal conductivity and were plotted versus temperature ( Fig. 3c ). Interestingly, the Lorentz number for the CNT–Cu composite linearly increased while remaining constant for Cu. Increasing Lorentz number indicates phonon contribution to the thermal conductivity, unlike a constant Lorentz number for a free electron system [42] . We extrapolated the Lorentz number at higher temperatures from the slope. The theoretically estimated ampacity was thus estimated as ∼ 1,200 MA cm −2 , which agrees with our measured ampacity of 600 MA cm −2 . These analyses and experimental results demonstrate the significant role of the CNT phonons in achieving high thermal conductivity and Lorentz number at elevated temperatures for the CNT–Cu composite. This phenomenon was vital for the high ampacity. Furthermore, we quantitatively evaluated the electromigration by estimating the Cu atomic fluxes in bulk Cu and CNT–Cu due to current (mass flux) described by the Nernst–Einstein equation [43] : where C is the concentration of atoms, k is the Boltzmann constant, T is the temperature, D * is the diffusion coefficient, F E and F T are the respective driving forces due to electron wind and temperature gradient. Electromigration consists of two components: the mass flux from electron wind (electron-Cu atom collisions, J E ) and from thermal gradient (diffusion caused by Joule heating, J T ). For Cu, the electron wind is known to be one order larger than that of the thermal gradient [44] ; thus, thermal gradient was neglected in the following discussion. We calculated the electron wind driving force by, where, z is the effective charge number [38] (=10), e the electronic charge (1.6 × 10 −19 C), ρ the material resistivity (4.3 × 10 −6 Ω cm), and j the current density (600 MA cm −2 ). By using experimentally obtained data, the electron-driving force was estimated to be (2,083 eV cm −1 ), two orders higher than that of Cu [44] (40 eV cm −1 ); accordingly, the electron wind mass flux was ∼ 100 times smaller than that of pure Cu. We think that this 100 times difference agrees well with the observed 100 times difference in ampacity. In summary, we developed a high-performance electrical conductor (CNT–Cu composite) that combines the best electrical properties of CNT (high ampacity) and Cu (high conductivity). Moreover, the CNT–Cu composite is the only material satisfying the ampacity and conductivity levels stipulated by ITRS [4] for 2015. Materials Single-walled CNTs were synthesized through the water-assisted supergrowth technique [34] . All chemicals were purchased from Wako and used without further purification, unless specified otherwise. Prefilling of CNT matrix with Cu electrolyte A free-standing CNT forest was obtained by carefully removing it from the growth substrate. This was subjected to a shear force between two glass slides to change the alignment direct of the CNT forest from vertical to horizontal (with reference to the glass slides). The arrangement, held in place using clips, was immersed into a densification solution of Copper acetate dissolved in acetonitrile (2.75 mM) and left undisturbed was 20 min. The densified solid was carefully removed and assembled into the electroplating setup. Electroplating setup The electroplating setup consists of a cathode of densified, prefilled CNT solid backed onto an stainless steel mesh for providing an equipotential surface for electroplating. The cathode was sandwiched between thin strips of pure Cu which served as anodes. Filter paper from Advantech acted as insulating separators between the anodes and cathode. The whole assembly was held in place using a specially designed polyether ether ketone cell. For the organic electroplating, the electrolyte consists of the same liquid, which was used during forest densification. In case of the second step aqueous electrodeposition, the electrolyte used was a commercially available electroplating solution (ATMI, without accelerators or suppressors). Trapped air and dissolved gases was removed from the setup before electrodeposition. Electrodeposition of Cu was carried out under galvanostatic conditions using a VMP3 Electrochemical workstation (Princeton Applied Research). Reductive annealing The composite after each electrodeposition was washed with pure acetonitrile and dried using a vacuum desiccator at 60 °C for 30 min. This was followed by heating at 250 °C for 3 h in a tube furnace. The heating and subsequent cooling was carried out under a controlled flow of H 2 gas at 150 sccm. Conductivity measurement The electrical conductivity measurements were carried out in two different geometries. The four-probe conductivity was measured using a hand-held four-probe conductivity meter fitted with Au-coated electrodes. For the two-probe measurement, the edges of the composite were cut using a CO 2 laser to remove the Cu deposited on the edges first removed to force the electrical path through the thickness (bulk) of the composite. Thin Cu strips were attached to either faces of the composite and were in turn connected to a digital multimeter. Plastic clips were used to hold the setup in place and ensure good, stable electrical contact between the electrodes and samples. Thus, the resistance measured was from the bulk of the composite, in a direction perpendicular to the thickness of the composite. The resistance of the composite was normalized to the thickness and cross-sectional area of the composite to arrive at its two-probe resistivity. The two-probe and four-probe conductivity values presented here are an average of five such measurements at different places of the composite across three composites. Microfabrication of CNT–Cu composite For microfabrication, vertically aligned CNT thin films were grown from patterned catalyst using water-assisted supergrowth chemical vapor deposition method. The average size of the films used here was 700 μm × 700 μm with an as-grown thickness of 8 μm. This was transferred to the desired substrate in the desired orientation using an liquid-induced densification approach [23] , [24] . Thickness of the CNT films after transfer was measured to be around 700 nm. Patterning of CNT film Ti-Au (3/100 nm) electrode lines, required during electrodeposition, were defined using conventional E-beam lithography followed by sputtering and lift-off. We used a TiN-coated Si 3 N 4 substrate to prevent Cu diffusion into the substrate, and large Ti/Au bottom contacts that ensured breakdown at the centre of the line. After CNT thin-film transfer, the substrate was vacuum baked at 180 °C for 15 min before resist coating. Positive tone PMMA-495 was spin-coated at 4,700 r.p.m. for 60 s on the substrate followed by baking at 180 °C for 60 s. This was followed by spin coating a negative tone FOX 16 resist at 4,500 r.p.m. for 60 s. The substrate was baked at 120 °C for 8 min for slow curing of the resist. E-beam lithography was used to define the required areas of CNT. The sample was developed using tetramethylammonium hydroxide, rinsed with water and dried under a dry N 2 flow. Reactive-ion etching using a mixture of O 2 /Ar /CHF 3 was carried out to remove the unwanted CNT areas. The negative resist was stripped by immersing in buffered hydrogen fluoride for ∼ 10 s followed by thorough rinsing and drying. The positive resist was removed using 1:1 micture of methylisobutyl ketone/isopropyl alcohol followed by rinsing in isopropyl alcohol and drying under N 2 stream. Current density testing of CNT–Cu composite A home-built setup was used to perform the current density testing on CNT–Cu composite. It consists of a T-joint fitted with electrical feedthrough on one side. The other two openings were connected to a vacuum pump and a vacuum gauge, respectively. All experiments were carried out at the pressure of 1.3 × 10 −4 Pa. The electrical feedthrough was connected to an Agilent U3606A DC power supply-Digital multimeter system capable of supplying up to 3 A. For higher currents, a Kikusui 10–105 DC power supply was used. The experiments were carried out by sequentially stepping up the voltage and simultaneously recording the current flowing through the system. Resistance at every voltage step, computed from the I–V correlation, was translated to resistivity with knowledge of length and cross-sectional area of the test structure. The cross-sectional area was also used to compute the applied current density at every stage of experiment. The testing was carried out on five devices with identical results. Sputtered and electroplated Cu films, Cu and Au wires (25 μm diameter), which are conventionally used in wire-bonding were also tested under identical conditions using the same setup. Activation energy analysis Accelerated lifetime tests were carried out at different temperatures using a modified setup consisting of a test chamber with temperature control. Electrical feedthrough in the test chamber enabled a constant current density to be applied while the temperature of the experiment could be modified. The time-to-failure of the sample at each temperature was recorded at a constant current density, providing an Arrhenius plot of ln(time-to-failure) versus 1/ kT . Activation energy for Cu diffusion in CNT–Cu composite was estimate from the slope of this graph. Lorentz number estimation Thermal diffusivity ( α ) of CNT–Cu composite was measured at various temperatures with a Bethel Thermowave Analyser system fitted with a temperature controller. Differential scanning calorimetry was used to estimate the specific heat capacity ( C p ) of the material in the same temperature range. Thermal conductivity ( κ ) of the sample at various temperatures was estimated using the relation where ρ is the density of the material (5.2 g cm −3 ). From the knowledge of electrical conductivity ( σ ) at various temperatures ( Fig. 1i ), the Lorentz number ( L ) was estimated using Wiedmann–Franz law as The Lorentz number estimated for Cu and CNT–Cu composite is plotted in Fig. 3c . How to cite this article : Subramaniam et al . One hundred fold increase in current carrying capacity in a carbon nanotube–copper composite. Nat. Commun. 4:2202 doi: 10.1038/ncomms3202 (2013).